Phase-locking to a free-space terahertz comb for metrological-grade terahertz lasers Optical frequency comb synthesizers have represented a revolutionary approach to frequency metrology, providing a grid of frequency references for any laser emitting within their spectral coverage. Extending the metrological features of optical frequency comb synthesizers to the terahertz domain would be a major breakthrough, due to the widespread range of accessible strategic applications and the availability of stable, high-power and widely tunable sources such as quantum cascade lasers. Here we demonstrate phase-locking of a 2.5 THz quantum cascade laser to a free-space comb, generated in a LiNbO 3 waveguide and covering the 0.1–6 THz frequency range. We show that even a small fraction (<100 nW) of the radiation emitted from the quantum cascade laser is sufficient to generate a beat note suitable for phase-locking to the comb, paving the way to novel metrological-grade terahertz applications, including high-resolution spectroscopy, manipulation of cold molecules, astronomy and telecommunications. Metrological-grade, high-power, terahertz sources offer great perspectives for applications in many different fields. Besides their straightforward use for high-resolution and high-sensitivity molecular gas spectroscopy [1] , [2] and far-infrared astronomy [3] , a number of disciplines could benefit from their actual availability. In biophysics, for example, narrow and stable terahertz radiation can help understand complex dynamics problems, in principle addressing high-precision molecular recognition and protein folding [4] . Similarly, absolute-frequency-controlled, high-power terahertz sources can be a key tool for controlling cold molecular ensembles [5] . Terahertz-emitting metrological sources, widely and continuously frequency-tunable, date back to the early 1980s [6] , [7] , and have recently evolved to systems based on photomixing techniques [8] , [9] . They are based on either microwave or infrared standards, ensuring a very high spectral purity and an absolute frequency reference, but a drawback is that their typical powers (above 1 THz) are at the nanowatt level. This has hindered, until now, the deployment of terahertz sources for experiments and applications requiring higher optical powers. In this context, extension of optical frequency comb synthesizers (FCSs) to the terahertz domain is a key progress. Optical FCSs have indeed represented a major improvement to frequency metrology [10] , [11] , separating the roles of light source and reference and providing, in principle, a frequency ruler for any laser emitting within their spectral range. Their huge potential is exploitable by directly beating the laser with one of the FCS teeth, and by detecting the beat note with a square-law detector. The test of maturity for frequency combs has been, indeed, the achievement of power levels suitable for an efficient detection of the beating signal with standard-grade detectors [12] . Several approaches have been recently pioneered to migrate the qualities of FCSs to the terahertz region. In a few cases, a link between a continuous wave (CW) terahertz source and a near-infrared comb has been provided by detection techniques based on photo-conductive antennas [13] or electro-optic crystals [14] . To detect and phase-lock the beat note, both these techniques involve the CW terahertz source in a low-efficiency up-conversion process. As a consequence, the CW-source power used for the phase-lock is larger than 1 mW. Such limitations can be overcome by producing a free-space terahertz FCS and by directly beating it with the CW terahertz source on a square-law detector. This experimental configuration allows independent optimization of the source and reference figures of merit, for an efficient beat-note detection. Once an appropriate detector is used, the amount of power needed for the frequency control of the terahertz source can be dramatically reduced, while making almost the whole power available for the experiment. The advent of terahertz quantum cascade lasers (QCLs) [15] is strongly motivating the development of terahertz metrological references. Indeed, as very recent studies have shown, QCLs exhibit a particularly high spectral purity (that is, narrow intrinsic linewidth) [16] , [17] , which further qualifies them as ideal metrological sources. On the other hand, although terahertz QCLs can presently deliver up to a few hundred milliwatt peak power at very low temperatures (10 K), a significant reduction of the output power levels is expected when temperatures > 150 K are approached [18] . From this perspective, the development of a power-efficient metrological referencing technique is therefore very promising. In this work, we demonstrate a free-space terahertz comb as a mature metrological tool. Indeed, we show that a 2.5 THz QCL can be directly beaten and phase-locked using a commercial hot-electron bolometer (HEB) detector, with only a few tens of nanowatt radiation power required. Terahertz FCS generation The presented terahertz FCS is based on a design commonly used for terahertz time-domain spectroscopy (TDS) [19] . In fact, regardless of the adopted emitter and configuration (antenna, crystal, etc. ), any pulsed source of this type is inherently a zero-offset terahertz FCS. Nevertheless, only recently the 'comb' nature of such sources has been recognized and exploited [20] , [21] , and no direct use of a terahertz comb as frequency 'ruler' for a terahertz laser has been reported so far. Our terahertz comb aims for a good trade-off between generation efficiency and spectral bandwidth. It is generated by optical rectification, based on the Cherenkov effect [22] , [23] of a femtosecond mode-locked Ti:sapphire laser in a waveguide fabricated on a MgO-doped LiNbO 3 crystal plate [24] , [25] . The single-mode linear waveguide, optimized for 800 nm wavelength propagation, is obtained by ion implantation onto the upper surface of the crystal plate. The generation scheme is sketched in Fig. 1a (see Methods for further details). The beam of the pump laser is focused into the waveguide by an aspheric lens. The waveguide lies just below one of the plate surfaces, thus minimizing absorption of the terahertz light within the crystal. We combined, in a non-standard approach, this linear waveguide design with a 45° high resistivity float zone silicon prism, in contact with the upper crystal surface, for efficiently extracting the train of terahertz pulses [26] . Each pulse consists of a single electric field cycle and carries a large spectral content, from 100 GHz up to 6 THz, centred at 1.6 THz ( Fig. 1b ). As the pulses are identical and equally spaced, the comb-like spectrum of the infinite train has a perfectly zero offset and a spacing corresponding to the 77.47 MHz repetition rate of the pump laser. In the best conditions, the average power of the generated terahertz radiation is of the order of 1 μW, as measured by a calibrated pyroelectric detector placed in front of the silicon prism. 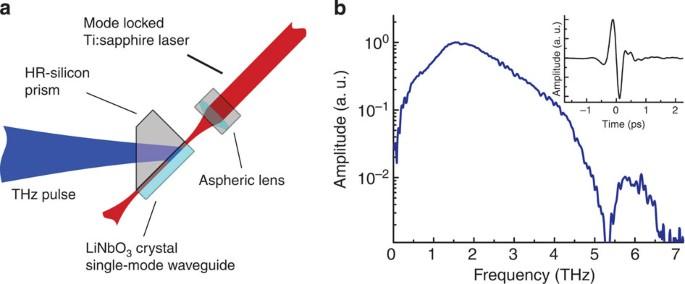Figure 1: Generation of the terahertz FCS. (a) Generation scheme of the terahertz pulses based on Cherenkov emission in a lithium niobate waveguide. (b) Terahertz comb spectral extension and single pulse temporal profile (inset) as measured with time-domain spectroscopy technique, using a photoconductive antenna as detector. The fast generation process, taking place in the LiNbO3crystal, enables extension of the frequency range up to 6 THz. The 'comb-like' feature arises from the repetition of identical pulses equally spaced in time. Figure 1: Generation of the terahertz FCS. ( a ) Generation scheme of the terahertz pulses based on Cherenkov emission in a lithium niobate waveguide. ( b ) Terahertz comb spectral extension and single pulse temporal profile (inset) as measured with time-domain spectroscopy technique, using a photoconductive antenna as detector. The fast generation process, taking place in the LiNbO 3 crystal, enables extension of the frequency range up to 6 THz. The 'comb-like' feature arises from the repetition of identical pulses equally spaced in time. Full size image Optical setup for beat-note detection and analysis We use a simple setup ( Fig. 2 ) and a commercial HEB detector to directly observe the beat note between individual comb teeth and a small fraction of the terahertz QCL emission. The QCL, emitting at a frequency around 2.5 THz (see Methods ), is housed in a liquid helium cryostat, and driven in continuous-wave mode at a fixed heat sink temperature T o ≈ 47.5 K. Under these experimental conditions the QCL threshold current is I th =375 mA, and the output power corresponding to the operating current I o =430 mA is P out ≈ 1 mW. 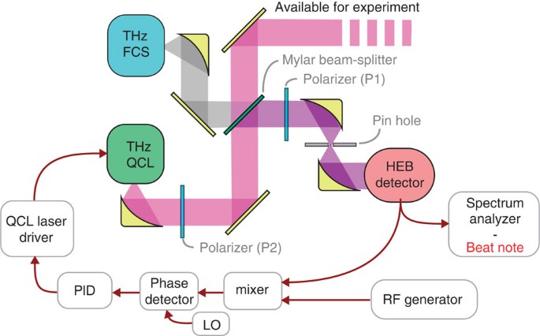Figure 2: Beat-note detection and phase-locking setup. The beating between the QCL and the FCS is detected on a HEB. The two beams are superimposed by means of a highly asymmetrical beam splitter, so that more than 99.5% of the QCL radiation is available for the experiment beam. The P1 polarizer ensures polarization matching between the beams, whereas P2 selects the amount of QCL power to be sent to the HEB. Indeed, the QCL terahertz radiation also works as local heater for the superconductive junction, bringing it at the suitable operating temperature. A sketch of the electronic setup is given in the lower part of the panel. The beat note is mixed with a synthesized RF signal, so that it is down-converted to the 21.4 MHz frequency of the phase-lock electronics local oscillator (LO). The output of the phase detector is processed by a standard proportional-integral-derivative (PID) unit and then sent to the QCL current driver, to close the locking loop. Figure 2: Beat-note detection and phase-locking setup. The beating between the QCL and the FCS is detected on a HEB. The two beams are superimposed by means of a highly asymmetrical beam splitter, so that more than 99.5% of the QCL radiation is available for the experiment beam. The P1 polarizer ensures polarization matching between the beams, whereas P2 selects the amount of QCL power to be sent to the HEB. Indeed, the QCL terahertz radiation also works as local heater for the superconductive junction, bringing it at the suitable operating temperature. A sketch of the electronic setup is given in the lower part of the panel. The beat note is mixed with a synthesized RF signal, so that it is down-converted to the 21.4 MHz frequency of the phase-lock electronics local oscillator (LO). The output of the phase detector is processed by a standard proportional-integral-derivative (PID) unit and then sent to the QCL current driver, to close the locking loop. Full size image Both the QCL and the pulsed terahertz beams were collected and collimated by 90° off-axis parabolic mirrors with an equivalent focal length of 25.4 mm. The two beams are then coupled by a mylar film which, at the given wavelength, works as an asymmetric beam splitter, so that most of the terahertz comb power and a small fraction of the QCL beam are overlapped and sent to the HEB. Optical coupling to the HEB is obtained by tuning collimation and diameter of the two beams by means of two 90° off-axis confocal parabolic mirrors. A pin hole, positioned in their focal plane, provides the required spatial mode cleaning, while a wire-grid polarizer ensures polarization matching. The optical powers of the QCL and the terahertz FCS impinging on the HEB have been measured by a calibrated pyroelectric detector. In the optimized conditions we have about 60 nW from the QCL beating with about 200 fW of the single comb tooth. Given the 70 fW noise-equivalent power (NEP) of the HEB, we expect a maximum beat note contrast of about 60 dB, in a 1 Hz bandwidth. The HEB 250 MHz electrical bandwidth (see Methods ) provides a wide frequency window where the beat note can be observed. In fact, as the spacing between the terahertz comb teeth is 77.47 MHz, there always are several beat notes falling within the detection bandwidth. This allows to detect higher-order beat notes, and gives the possibility to select the Fourier interval where a lower background noise maximizes the signal-to-noise ratio. The signal obtained from the HEB detector is split and sent to a fast Fourier transform (FFT) real-time spectrum analyser (see Methods for further details) for the beat-note measurements, and to the phase-lock electronics. A typical FFT spectrum of the detected signal is shown in Fig. 3a , together with a schematic sketch of the observed frequencies. The spectrum shows both a pair of peaks spaced by 77.47 MHz, arising from the beating of comb teeth among themselves, and a pair of smaller peaks, generated by the beating of the QCL with two distinct comb teeth, one at its left and one at its right. In the case shown, they correspond to the beating with the third-order neighbours teeth. Once the order of the involved comb tooth is known, the measurement of the beat-note frequency can be used to retrieve the QCL absolute frequency, thus enabling to count it and to trace its temporal evolution in real time. 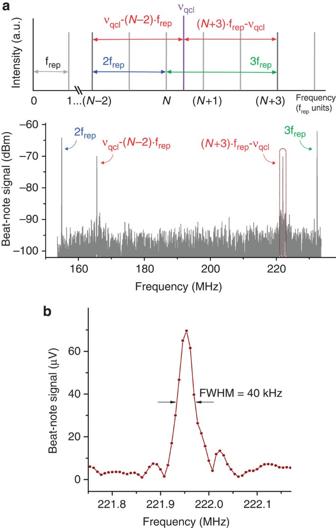Figure 3: Beat-note detection. (a) The upper sketch shows, in the frequency domain, the comb-like structure of the terahertz FCS beam, as well as the monochromatic QCL emission (νqcl). The red-coloured arrows indicate the beating between the QCL and the third-order neighbours teeth of the comb. The corresponding frequencies fall in the range between 2frepand 3frep(blue and green arrows, respectively), and are shown in the FFT spectrum below, together with the self-beatings among the comb teeth (as highlighted by the coloured labels). The beat-note frequency is given, apart from frepmultiples, by its distance from the closestNthand (N+1)thteeth of the comb. Therefore, once the orderNis known, the QCL absolute frequency can be retrieved. (b) Zoomed view of the beat-note peak around 222 MHz (dashed box ina), acquired with a 20 kHz RBW. The 40 kHz FWHM gives the emission linewidth of the free-running QCL over 1 ms observation time. Figure 3: Beat-note detection. ( a ) The upper sketch shows, in the frequency domain, the comb-like structure of the terahertz FCS beam, as well as the monochromatic QCL emission (ν qcl ). The red-coloured arrows indicate the beating between the QCL and the third-order neighbours teeth of the comb. The corresponding frequencies fall in the range between 2f rep and 3f rep (blue and green arrows, respectively), and are shown in the FFT spectrum below, together with the self-beatings among the comb teeth (as highlighted by the coloured labels). The beat-note frequency is given, apart from f rep multiples, by its distance from the closest N th and ( N +1) th teeth of the comb. Therefore, once the order N is known, the QCL absolute frequency can be retrieved. ( b ) Zoomed view of the beat-note peak around 222 MHz (dashed box in a ), acquired with a 20 kHz RBW. The 40 kHz FWHM gives the emission linewidth of the free-running QCL over 1 ms observation time. Full size image The FFT spectrum analyzer is also used to retrieve the width of the beat note at different timescales. Figure 3b shows the beat-note peak over a single FFT spectrum acquisition time (1 ms). The measured full width half maximum (FWHM) of about 40 kHz is in good agreement with previous independent results [27] , [28] and with our previous measurements of the frequency-noise power spectral density of the same device [17] . It provides a quantitative estimation of the spectral purity of the laser emission over a 1 ms timescale, whereas on longer timescales the jitter of the QCL frequency obviously leads to broader signals. 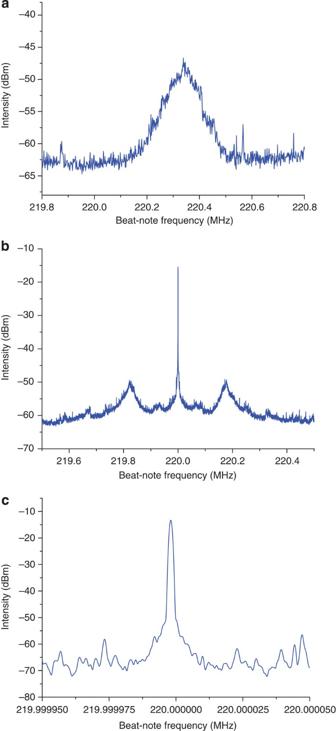Figure 4: FFT spectrum analyzer acquisition spectra. The lineshape of the beat-note spectra gives direct evidence of the effects of the phase-lock on the QCL emission. (a) Unlocked QCL, with 1 MHz span and 100 Hz RBW. (b) Phase-locked beat-note signal acquired with a 1 MHz span and 100 Hz RBW. The two sidebands indicate a phase-lock electronic bandwidth of about 200 kHz. (c) Phase-locked beat-note signal acquired with a 100 Hz span and 1 Hz RBW. Figure 4a shows the 250 kHz FWHM of the free-running beat note, analysed over a 100 ms timescale. Figure 4: FFT spectrum analyzer acquisition spectra. The lineshape of the beat-note spectra gives direct evidence of the effects of the phase-lock on the QCL emission. ( a ) Unlocked QCL, with 1 MHz span and 100 Hz RBW. ( b ) Phase-locked beat-note signal acquired with a 1 MHz span and 100 Hz RBW. The two sidebands indicate a phase-lock electronic bandwidth of about 200 kHz. ( c ) Phase-locked beat-note signal acquired with a 100 Hz span and 1 Hz RBW. Full size image Phase-lock between terahertz QCL and FCS To effectively stabilize the phase of the QCL emission to the frequency comb reference, a phase-lock loop (PLL) has been implemented. The simplified scheme of the electronic setup used for closing the PLL is given in Fig. 2 . The beat-note signal is mixed with a synthesized fixed frequency and processed by an analog/digital phase detector. The correction signal closes the PLL on the fast (1 MHz bandwidth) modulation input of our home-made low-noise QCL current driver. Locked beat-note spectra at different spans and resolution bandwidths (RBWs) are shown in Fig. 4b,c . The electronic bandwidth of the loop is about 200 kHz, and the achieved signal-to-noise ratio is >50 dB at 1 Hz RBW, close to the expected limit of 60 dB. By numerical integration of the beat-note spectra, we find that about 75% of the QCL power is phase-locked to the FCS emission. The phase-lock leads to a narrowing of most of the CW laser emission down to the terahertz comb tooth linewidth. As shown by Yasui et al . [20] , the linewidth of a terahertz photo-carrier comb (at 100 GHz) is just few hertz wide (in 1 s). Similar results can be achieved by our system, once proper stabilization of the pump laser repetition rate is set. Beyond the observed performances, ample room is left for additional improvements to further enhance the beat-note signal-to-noise ratio. One relies on proper spectral filtering of the broad-band terahertz FCS that would reduce the portion of power contributing to noise but not to the beating. The second is the optimization of the comb generation process. In particular, a chirped waveguide design can be developed to compensate pump pulse dispersion along its propagation, thus increasing the crystal volume involved in generation. Moreover, the development of new high-bandwidth, low-NEP, terahertz detectors, such as nanowire field-effect transistors [29] , [30] , could bring, in the next future, to a room-temperature detection of the beat-note signal. In conclusion, we demonstrate phase locking of a 2.5 THz QCL to a 6-octaves frequency-spanning air-propagating terahertz FCS. The CW terahertz power required for the phase-lock is four orders of magnitude lower than in other previous approaches. The proposed technique will therefore have a key role in experiments where only a negligible fraction of the terahertz source power is available for phase/frequency control. This paves the way to new experiments and applications in the terahertz range, such as absolute frequency measurements of sub-Doppler molecular spectra, phase locking of high-temperature terahertz QCLs, or manipulation and control of cold molecules. Crystal plate design The MgO-doped LiNbO 3 crystal plate, purchased from the HC-Photonics company, has the dimensions of 8×10×0.5 mm 3 . It holds two linear waveguides, obtained by ion implantation on the same crystal surface, oriented along the 10 mm-long side. Their design is optimized for single-mode propagation of a 800 nm radiation, with an effective mode size of about 5 μm diameter. According to the Cherenkov configuration, the orientations of the optical field polarization and the crystal optical axis have been chosen both parallel to the crystal plate surface and orthogonal to the waveguide input surface. This choice allows the maximization of the terahertz emission outgoing from the plate surfaces. Pump laser source The pump laser is a self-mode-locked Ti:sapphire laser (by Femtolasers, mod. Fusion) emitting pulses with 25 fs temporal width, 77.47 MHz repetition rate, around 800 nm wavelength. As the repetition rate is not stabilized, it is affected by slow drifts of the order of hundreds of millihertz in 1 s. This instability does not affect the measurements discussed in the paper, as the observation time of the beat note is much shorter than 1 s. HEB detector The commercial detector used for the beat-note acquisition is a HEB detector by Scontel, model RS 0.3–3T-1, whose sensitive element is a 6 nm-thick MoRe bridge. The active area of the sensitive element is connected to a log-spiral antenna, whose main lobe is coupled with a silicon lens. The HEB chip and the lens are mounted on the bolometer holder of a liquid helium cryostat, while the signal radiation is received through a high density polyethylene window. A low-noise cryogenic amplifier, with a 250 MHz bandwidth, is housed inside the same cryostat. Its output signal is directly processed by our real-time spectrum analyzer (see below). A local heater is used for keeping the HEB temperature just below the superconductive transition of the junction. During all the measurements presented in this paper, however, the local heater is switched off, as the QCL radiation itself works as local heater. To allow a fine regulation of the QCL intensity and, consequently, of the HEB junction temperature, a second polarizer has been added along the QCL beam path (labelled as P2 in Fig. 2 ). Real-time spectrum analysis The spectral analysis of the beat-note signal is carried out by a real-time spectrum analyzer (Tektronix, model RSA5106A). The signal, in the time domain, is digitized at 14 bits and at a 300 Ms s −1 sampling rate. A FFT operation is then applied to consecutive sets of the temporal trace, thus allowing to reconstruct the temporal evolution of the signal spectrum. QCL fabrication procedure The investigated device is a QCL operating at 2.5 THz and based on a bound-to-continuum design. The heterostructure has been grown by molecular beam epitaxy employing a GaAs/Al 0.15 Ga 0.85 As heterostructure [14] on a nominally undoped GaAs substrate. The waveguide core is formed by 110 repetitions of the gain medium that creates a 14 μm thick active region, while the confinement of the emitted light is ensured by a buried highly doped GaAs layer with negative dielectric constant. Devices were processed into 150 μm wide laser ridges by optical lithography, with ohmic contact deposition and with a standard surface-plasmon waveguide [14] . Lateral contacts to the buried highly doped layer were kept 30 μm away from the ridge side, to avoid too much coupling with the optical mode. The waveguide was completed by the evaporation of Cr/Au on top of the ridge to create the main surface–plasmon interface. The lasers were then soldered to a copper bar, wire bonded and mounted on the cold finger of a liquid helium cryostat. How to cite this article: Consolino, L. et al . Phase-locking to a free-space terahertz comb for metrological-grade terahertz lasers. Nat. Commun. 3:1040 doi: 10.1038/ncomms2048 (2012).